Nitrogen-doped carbon nanomaterials as non-metal electrocatalysts for water oxidation Efficient and low-cost electrocatalysts for the oxygen evolution reaction are essential components of renewable energy technologies, such as solar fuel synthesis and providing a hydrogen source for powering fuel cells. Here we report that the nitrogen-doped carbon materials function as the efficient oxygen evolution electrocatalysts. In alkaline media, the material generated a current density of 10 mA cm −2 at the overpotential of 0.38 V, values that are comparable to those of iridium and cobalt oxide catalysts and are the best among the non-metal oxygen evolution electrocatalyst. The electrochemical and physical studies indicate that the high oxygen evolution activity of the nitrogen/carbon materials is from the pyridinic-nitrogen- or/and quaternary-nitrogen-related active sites. Our findings suggest that the non-metal catalysts will be a potential alternative to the use of transition metal-based oxygen evolution catalysts. The impending global energy crisis has prompted intense research into the development of various types of sustainable energy conversion and storage systems [1] . In particular, water splitting, by either electrochemical or photo-electrochemical reactions, is a practical and environmentally friendly approach to generate hydrogen for powering fuel cells and reduce CO 2 to fuels [2] , [3] , [4] , [5] . However, the efficiency of electrochemical water splitting is limited by the considerable overpotential requirement of the reaction [6] and the need for expensive noble metal catalysts, such as iridium and ruthenium oxides [7] , [8] , [9] , [10] . Thus, it is important to discover efficient and cost-effective electrocatalysts for the oxygen evolution reaction (OER) [11] . In natural photosynthetic systems, cubane-like calcium manganese cluster (CaMn 4 O 5 ) complexes function as an OER catalyst for effective solar fuel synthesis [12] . Consequently, researchers have attempted to biomimic natural compounds, such as hybrids of CaMn 2 O 4 and Mn 3 O 4 /CoSe 2 , to obtain efficient OER electrocatalysts [13] , [14] , [15] . However, a nanocomposite of Mn 3 O 4 /CoSe 2 required an overpotential of approximately 0.45 V in potassium hydroxide (KOH) solution (pH 13) to achieve a current density of 10 mA cm −2 (current density based on geometric surface area (GSA)) [15] . Other studies have also attempted to use non-precious metal oxide materials/structures, such as perovskite [6] , [16] , and cobalt [17] , [18] and manganese oxides and their derivatives [19] , [20] , [21] , to replace noble metal materials for the OER process. A high OER activity of a low-cost catalyst was achieved in an alkaline electrolyte (pH 14) using a Co 3 O 4 /N-graphene synergistic catalyst, which generated a current density of 10 mA cm −2 at an overpotential of approximately 0.4 V [11] . Most recent efforts to construct efficient and low-cost OER electrocatalysts have mainly focused on transition metal oxide-based catalysts, as metal species are widely regarded to be the active sites for electrochemical OER. However, the use of state-of-the-art electrocatalysts is complicated by the complex preparation methods and low electrical conductivity of transition metal oxides, and the catalytic performance remains unsatisfactory. Thus, novel and sophisticated strategies for material synthesis are required for achieving cost-effective OER catalysts with low overpotentials. Very recently, N (5)-ethyl-flavinium ions were found to function as organic non-metal electrocatalysts for water oxidation by mediating a four-electron transfer reaction [22] . Although a much higher overpotential is required for this electrocatalyst (0.73 V versus reversible hydrogen electrode (RHE), pH 2) compared with existing transition metal-based catalysts, this work has opened up a new category of OER electrocatalysts. However, the next challenge is to improve the catalytic activity of such a non-metal electrocatalysts for overcoming the limitation of the existing transition metal-based OER electrocatlysts. Here we demonstrate that nitrogen-doped graphite nanomaterials synthesized from a nitrogen-rich polymer exhibit highly efficient OER activity in alkaline media exceeding those of traditional electrocatalysts. Notably, in the absence of transition metals, the optimized nitrogen/carbon materials show OER overpotentials as low as 0.38 V at a current density of 10 mA cm −2 in pH 13 medium, which is the best among the non-metal OER electrocatalysts. Detailed electrochemical and physical studies indicate that the high OER activity of the nitrogen/carbon materials is from the pyridinic-N- or/and quaternary-N-related active sites. The concept of the non-metal electrocatalyst is further identified using nitrogen-contained graphene materials for OER process. The preparation and OER activity of the nitrogen-doped carbon materials The nitrogen-doped carbon (N/C) materials used in this study were synthesized by pyrolysing the hybrid of a melamine/formaldehyde polymer and nickel nitrate at 700 °C ( Fig. 1 ) (ref. 23 ). Concentrated hydrochloride acid was then added to remove the metal species from the N/C material. A sample of pyrolysed N/C material that was not subjected to acid leaching was also prepared for a reference and was termed N/C–NiO x in this work. After obtaining powder samples of N/C and N/C–NiO x , film electrodes were prepared using a catalyst/nafion-polymer ink to deposit the synthesized materials on a glassy carbon electrode in a rotating ring-disk electrode (RRDE) system for electrochemical characterization. 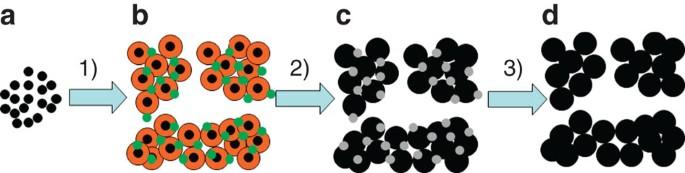Figure 1:Synthesis procedure of the N/C materials. Steps: (1) synthesis of melamine formaldehyde (MF) polymer with nickel nitrate and carbon particles; (2) pyrolysing metal-salt/MF-polymer precursor; and (3) acid leaching of the pyrolysed samples. Materials: (a) carbon particles (black dot); (b) carbon particles covered with MF polymer (yellow sphere) and nickel nitrate (green dot); (c) N/C–NiOxcatalyst (grey dot, NiOx); and (d) N/C catalyst. Figure 1: Synthesis procedure of the N/C materials . Steps: (1) synthesis of melamine formaldehyde (MF) polymer with nickel nitrate and carbon particles; (2) pyrolysing metal-salt/MF-polymer precursor; and (3) acid leaching of the pyrolysed samples. Materials: ( a ) carbon particles (black dot); ( b ) carbon particles covered with MF polymer (yellow sphere) and nickel nitrate (green dot); ( c ) N/C–NiO x catalyst (grey dot, NiO x ); and ( d ) N/C catalyst. Full size image The OER activity of the N/C materials was assessed using a RRDE system in which a glassy carbon electrode, Pt wire and saturated calomel electrode (SCE) served as the working, counter and reference electrodes, respectively. N/C–NiO x , IrO 2 /C (20 wt%) [24] (scanning electron microscopy (SEM) image of IrO 2 /C ( Supplementary Fig. S1 ) and BET surface area ( Supplementary Table S1 ) are provided) and commercial Pt/C (20 wt%, 600 m 2 g −1 ) were used as reference catalysts to compare their OER activities with that of N/C. Optimized N/C catalysts (N/C pyrolysed at 700 °C) were used in experiments unless otherwise specified. Cyclic voltammetry (CV) was performed in a KOH solution (pH 13) at 25 °C with a sweep rate of 5 mV s −1 and an RDE rotation speed of 1,500 r.p.m. The calculation of current density at 10 mA cm −2 for the OER activity was based on the GSA unless otherwise specified, which was commonly used for characterizing the OER activity of electrocatalysts in research community [11] , [15] , [19] , [20] , [21] . As shown in Fig. 2a , the N/C catalyst generated a current density of 10 mA cm −2 at a potential of 1.61±0.01 V versus RHE (mean±s.d., n =5), which is similar to that of IrO 2 /C materials (10 mA cm −2 , 1.60±0.01 V). The electrochemical active surface area (EASA) of N/C and IrO 2 /C (20 wt%) materials are measured, and their values are close ( Supplementary Table S1 ), demonstrating that their OER activities are also similar based on the EASA. With the employed sweep rate (5 mV s −1 ), the forward and backward scans almost overlapped for the N/C electrodes, indicating that the capacitive current was very low ( Supplementary Fig. S2 ). The amount of evolved oxygen was monitored simultaneously with current density ( J ) versus potential ( V ) measurements using a needle-type oxygen microsensor. The evolved O 2 gas was detected at an onset potential of 1.52±0.02 V versus RHE ( Fig. 2b ), clearly showing that the N/C catalyst has OER activity. 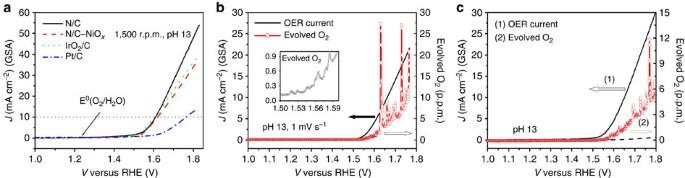Figure 2: OER activities of the different electrocatalysts. (a) Oxygen evolution activities of the N/C, N/C–NiOx, IrO2/C (20 wt%) and Pt/C (20 wt%) electrodes with KOH electrolyte (pH 13) analysed from RRDE system (loading catalyst: 0.2 mg cm−1; rotation speed: 1,500 r.p.m.; and scan rate: 5 mV s−1). (b) The amount of evolved O2(curve 1) and current density on the N/C electrode (curve 2) during the positive potential sweep with the electrochemical cell (inset: the evolved O2in the potential range from 1.5 to 1.6 V) working electrode, graphite carbon; reference electrode, Ag/AgCl/KCl, counter electrode, Pt wire, 0.1 mg cm−2N/C catalyst, scan rate, 1 mV s−1. (c) OER activity of the pyrolysed graphene/PDPS analysed from RRDE system (curve 1, solid line, test similar asFig. 2a) and the evolved O2on the pyrolysed graphene/PDPS electrode with the electrochemical cell (curve 2, test similar asFig. 2b). (Dash line, pure graphene electrode.) Figure 2: OER activities of the different electrocatalysts. ( a ) Oxygen evolution activities of the N/C, N/C–NiO x , IrO 2 /C (20 wt%) and Pt/C (20 wt%) electrodes with KOH electrolyte (pH 13) analysed from RRDE system (loading catalyst: 0.2 mg cm −1 ; rotation speed: 1,500 r.p.m. ; and scan rate: 5 mV s −1 ). ( b ) The amount of evolved O 2 (curve 1) and current density on the N/C electrode (curve 2) during the positive potential sweep with the electrochemical cell (inset: the evolved O 2 in the potential range from 1.5 to 1.6 V) working electrode, graphite carbon; reference electrode, Ag/AgCl/KCl, counter electrode, Pt wire, 0.1 mg cm −2 N/C catalyst, scan rate, 1 mV s −1 . ( c ) OER activity of the pyrolysed graphene/PDPS analysed from RRDE system (curve 1, solid line, test similar as Fig. 2a ) and the evolved O 2 on the pyrolysed graphene/PDPS electrode with the electrochemical cell (curve 2, test similar as Fig. 2b ). (Dash line, pure graphene electrode.) Full size image The OER overpotentials at a current density of 10 mA cm −2 were comparable to the performance of other reported OER catalysts, including Co 3 O 4 /N-graphene (1.63 V versus RHE, pH 14) (ref. 11 ), Mn 3 O 4 /CoSe 2 hybrids (1.68 V versus RHE, pH 13) (ref. 15 ) and IrO 2 nanoparticles (1.7 V versus RHE, pH 13) (ref. 7 ). Although the N/C–NiO x catalyst required a potential of ~1.65±0.01 V to obtain a current density of 10 mA cm −2 (GSA), the calculated OER activity of the N/C–NiO x based on the EASA ( Supplementary Table S1 ) was comparable to that of the N/C materials ( Supplementary Fig. S3 ). For Pt/C (20 wt%) catalysts, the potential required to generate a current density of 10 mA cm −2 was ~1.73±0.02 V, roughly 0.1 V higher than that of the N/C catalyst. Amperometric responses of Pt ring electrodes at a constant potential of 1.51 V in the RRDE system were also monitored for detecting peroxide species formed at the N/C catalyst surface of the disk electrode by following the literature method. [22] As shown in Supplementary Fig. S4 , almost no hydrogen peroxide was detected on the ring electrode at a scan potential ranging from 1.0 to 1.8 V (versus RHE), suggesting that the N/C catalyst favoured the four-electron oxidation of water. Physical characterization of the N/C materials To investigate the properties of the N/C material, X-ray diffraction (XRD), SEM and transmission electron microscopy (TEM) were performed. Supplementary Fig. S5 shows the XRD spectra of the N/C and N/C–NiO x samples. The peaks at 2 θ =26.4 o and 2 θ =44 o correspond to the (002) plane of the graphite structure and the (100) plane of the disordered amorphous carbon, respectively [25] . The observed peaks indicate that the N/C materials are graphite-based materials. The XRD peaks of the N/C–NiO x sample indicate that it contains nickel/nickel oxide compounds [26] , [27] (a carbon peak was not observed in the spectrum because of the much lower carbon peak intensity than that of nickel species). 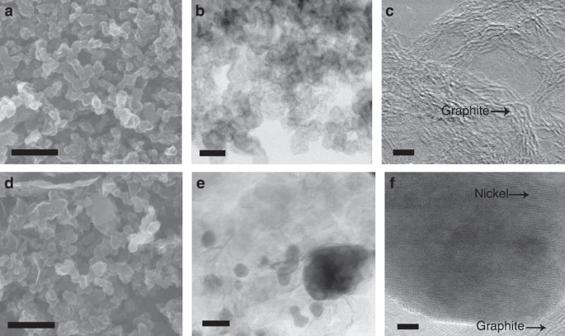Figure 3: SEM and TEM images of the N/C and N/C–NiOxmaterials. (a–c) The N/C samples. (d–f) The N/C–NiOxsamples. Scale bar, 250 nm (a,d); 50 nm (b,e); and 2 nm (c,f). Nickel species are found to be existed or not in the N/C and N/C–NiOxgraphite nanomaterials, respectively. Figure 3 shows the SEM ( Fig. 3a,d ) and TEM images ( Fig. 3b,c,e,f ) of the N/C ( Fig. 3a–c ) and N/C–NiO x ( Fig. 3d–f ) catalysts. From the SEM images, the diameter of the N/C catalyst was determined to be approximately 30–40 nm ( Fig. 3a ). TEM images of the N/C catalysts confirmed the estimated size of the catalyst, and no metal particles were observed in the N/C samples ( Fig. 3b ). SEM imaging of the N/C–NiO x catalyst revealed that several clusters of large particles had formed and were ascribed to the nickel species in the N/C–NiO x samples ( Fig. 3d ). The TEM images of N/C–NiO x ( Fig. 3e ) confirmed that nickel oxide particles were distributed in the sample. High-resolution TEM images showed that the N/C ( Fig. 3c ) and N/C–NiO x ( Fig. 3f ) samples were graphite-based nanomaterials, and that the nickel oxide crystals were surrounded by layered graphite in the N/C–NiO x materials. Figure 3: SEM and TEM images of the N/C and N/C–NiO x materials. ( a – c ) The N/C samples. ( d – f ) The N/C–NiO x samples. Scale bar, 250 nm ( a , d ); 50 nm ( b , e ); and 2 nm ( c , f ). Nickel species are found to be existed or not in the N/C and N/C–NiO x graphite nanomaterials, respectively. Full size image Energy dispersive spectroscopy (EDS)–TEM was performed to confirm the observed elemental distribution of the N/C and N/C–NiO x samples ( Supplementary Fig. S6 ). Uniform distribution of C, N and O elements was found in both the N/C and N/C–NiO x samples by determination of the X-ray map in the EDS–TEM analysis, whereas the nickel species were detected only in the N/C–NiO x sample. The test of elemental content in the N/C and N/C–NiO x samples by EDS–TEM also showed that no nickel species were present in the N/C materials ( Supplementary Fig. S7 , the detection limit of EDS–TEM system: 0.05–0.1 at%). This finding contrasts with those of iron- and cobalt-derived N/C materials, in which small amount of metal particles were still observed after long-duration pyrolysis and acid hydrolysis [28] . It was possibly ascribed to the as-used melamine/formaldehyde resin and nickel precursors, resulting in that the nickel species were hardly bound to the carbon matrix after pyrolysation and strong acid leaching. It strongly suggests to us that the OER activities of the N/C materials are due to the nitrogen-related active sites. We confirmed that nickel species cannot be detected by X-ray photoelectron spectroscopy (XPS) for the N/C material; C: 93.5%, N: 4.1%, O: 3.1% and Ni: 0.0% ( Supplementary Fig. S8 , the detection limit of the XPS: 0.05–0.1 at%). Elemental analysis of the possible metal species existed in the N/C catalyst (700 °C) was further conducted using inductively coupled plasma-atomic emission spectroscopy (ICP-AES). The detected concentration of Ni was 0.002 at%, indicating that the amount of metal Ni was negligible (see also the detailed discussion in Methods). The OER activity of the pyrolysed graphene/poly(bis-2,6-diaminopyridinesulphoxide) catalyst Thus, the above results indicated that the N/C material did not contain nickel species, although nickel was used during the synthesis of the material. To completely exclude the possibility that trace amount of nickel serves as the active reaction centre, a new N/C material was synthesized from pyrolysing the hybrids of graphene oxide and poly(bis-2,6-diaminopyridinesulphoxide) (PDPS, nitrogen-rich polymer) at 900 °C for 5 min [29] , [30] . None of the transition metals was introduced even during the synthesis process of the pyrolysed PDPS/graphene sample, which can totally exclude the possible contribution of metals on the OER activity. The SEM image of pyrolysed graphene/PDPS (Supplementary Fig. S9) showed the layered structure, and the BET surface area of the pyrolysed PDPS/graphene materials was 214 m 2 g −1 . The pyridinic-N (56.5%) and quaternary-N (37.4%) were the dominant species in the nitrogen states of the PDPS/graphene samples ( Supplementary Fig. S9 ). The pure graphene electrode did not show the OER activity at the scanned potentials (dash line in Fig. 2c ), whereas the pyrolysed graphene/PDPS demonstrated a current density of 10 mA cm −2 (GSA) at 1.64±0.01 V (curve 1, solid line in Fig. 2c ), which was a little higher that of the N/C materials (10 mA cm −2 , 1.61±0.01 V). The evolved O 2 gas could be also detected by the oxygen sensor used in the previous electrochemical cell (curve 2). It proved that nitrogen-related active sites can serve for the high OER activity. The N-content (1.7 wt%) and specific surface area (214 m 2 g −1 ) of PDPS/graphene were lower than those of the N/C materials (4.1 wt%, 560 m 2 g −1 ), respectively ( Supplementary Tables S1–S3 ). It was the reason that the resultant OER activity was a little lower than that of the N/C materials. The catalytic OER active sites of the N/C materials Next, we tried to identify the catalytic OER active sites. As it is known that heteroatoms, such as nitrogen atoms, escape from the carbon matrix during the pyrolysis process [31] . Therefore, the N/C catalysts with different concentrations of nitrogen can be obtained by adjusting the pyrolysis temperature, thereby facilitating investigation of the effects of nitrogen on OER activity. As shown in Fig. 4 , increasing the pyrolysis temperature to 700–1,000 °C resulted in a positive shift of the OER overpotential, with 700 °C being the optimal temperature for the highest yield of OER catalysts. The EASA and BET surface area of the N/C materials pyrolysed at different temperatures were also measured to compare their catalytic activity based on actual surface area ( Supplementary Table S1 , the calculation of EASA was based on the relationship between the capacitors and the loaded catalyst amount and shown in Methods and Supplementary Fig. S10 ). The EASA and BET surface area were slightly increased after increase of the pyrolysation temperatures (from 17.5 to 18.5 cm 2 ; electrode GSA, 0.2 cm 2 , Supplementary Table S1 ). Because of the low electrical resistivity of the N/C material pyrolysed at 600 °C (1.7 × 10 2 Ω cm), it showed much lower OER activities than that of the N/C catalyst pyrolysed at 700 °C (8.5 × 10 −1 Ω cm). 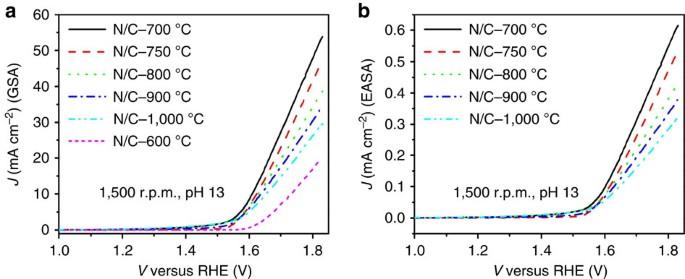Figure 4: OER activities of the different N/C catalysts. The OER activities were evaluated according to (a) GSA and (b) EASA. The best N/C catalyst synthesized at 700oC exhibited a current density of 10 mA cm−2(GSA) at a lowest OER overpotential (loading catalyst: 0.2 mg cm−1; rotation speed, 1,500 r.p.m.; and scan rate: 5 mV s−1). Figure 4: OER activities of the different N/C catalysts. The OER activities were evaluated according to ( a ) GSA and ( b ) EASA. The best N/C catalyst synthesized at 700 o C exhibited a current density of 10 mA cm −2 (GSA) at a lowest OER overpotential (loading catalyst: 0.2 mg cm −1 ; rotation speed, 1,500 r.p.m. ; and scan rate: 5 mV s −1 ). Full size image XPS was used to study the elemental state of the N/C catalyst surface. Supplementary Table S2 summarizes the surface elemental composition of the N/C–NiO x and N/C catalysts pyrolysed at different temperatures. As the N/C catalyst pyrolysed at 600 °C exhibited high electrical resistivity (1.7 × 10 2 Ω cm), it was not used as a reference sample for the comparison of OER activities. The XPS analysis revealed that the nitrogen concentration of the N/C materials gradually decreased with increasing pyrolysis temperature (in the range of 700–1,000 °C). For the N/C samples pyrolysed at 700 and 750 °C, no metal species were detected by XPS; however, when the pyrolysis temperature was increased to 800–1,000 °C, a low level of nickel species was detected. We speculate that a trace amount of nickel species is trapped inside of the carbon matrix and does not leach from the N/C samples during acid hydrolysis. For the N/C catalysts, the N1s XPS spectra were deconvoluted into three peaks (pyridinic-N, 398.4 eV; quaternary-N, 400.6 eV; and pyridinic-N + -O − , 403.8 eV) according to their binding energies ( Fig. 5a ) [32] , [33] . The pyridinic-N (54.8%) and quaternary-N (37.0%) were the dominant species in the nitrogen states of the N/C samples ( Supplementary Fig. S11 ; Supplementary Tables S4 and S5 ). We also examined the relationship between the amount of total nitrogen, nitrogen species and nickel metal in the N/C (700 °C) sample and the OER activity (the defined OER activity was based on the calculation of current density at 1.60 V from the EASA, Fig. 5b ). With increasing levels of pyridinic-N and quaternary-N, the OER activity of the N/C catalyst improved. No clear relationship was detected between the nickel and quaternary-N + -O − species, and the OER activity, which strongly suggests that nitrogen-related species is the active centre of OER activity. 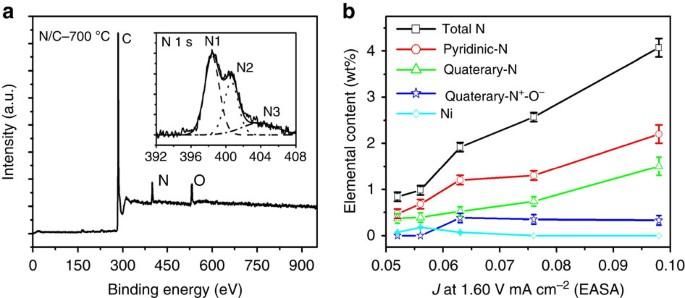Figure 5: XPS spectra and activity parameters of the N/C materials. (a) XPS spectra of the N/C materials prepared at 700 °C. Inset shows a high-resolution deconvoluted N 1 s spectrum. (N1: pyridinic-N, N2: quaternary-N and N3: quaternary-N+-O−) (b) Relationship between the different elemental contents and OER activities of the N/C electrocatalyst (the potentials required to achieve 10 mA cm−2). The calculated current density is based on the EASA. The concentrations of pyridinc-N and quaternary-N are positively correlated with the OER activities. Figure 5: XPS spectra and activity parameters of the N/C materials. ( a ) XPS spectra of the N/C materials prepared at 700 °C. Inset shows a high-resolution deconvoluted N 1 s spectrum. (N1: pyridinic-N, N2: quaternary-N and N3: quaternary-N + -O − ) ( b ) Relationship between the different elemental contents and OER activities of the N/C electrocatalyst (the potentials required to achieve 10 mA cm −2 ). The calculated current density is based on the EASA. The concentrations of pyridinc-N and quaternary-N are positively correlated with the OER activities. Full size image The OER stability of the N/C materials To evaluate OER stabilities of the N/C catalysts, continuous CV in the RDE tests was performed in KOH solutions (pH 13). As shown in Supplementary Fig. S12 , OER catalytic current of N/C electrode at the 20th sweep was almost the same as that at the first sweep, proving the activity stability of N/C catalyst. As a large amount of O 2 was evolved in the pores of N/C electrodes during OER process and the catalyst layer was peeled off from the glassy carbon electrodes, the decreased catalytic activity after the 20th sweep was possibly from the physical loss of the N/C catalysts, the instability of nafion-polymer binder or instability of the N/C materials. The clear instability mechanism and the improvement of the OER stability are now under investigation. In the aforementioned results, the OER activities of the N/C materials are considered to stem from the nitrogen-related species. As OER is a reverse reaction of ORR, we think that OER active sites of the N/C materials are similar to those of N/C catalysts for ORR in the previous reports [34] , [35] , [36] , [37] . At the first step, carbon atoms adjacent to nitrogen atoms are positively charged because of the electron-withdrawing nitrogen atoms in a graphene π-system [34] . Positively charged carbon around nitrogen to absorb OH − can be easily understood. For the limited step of OER, one of the possible explanations is that the neighbouring positive-charged carbon atoms support the easy recombination of two O ads additives [2] , [30] , [35] . Another possible mechanism may be from nitrogen atoms. As the density of state of nitrogen in a graphitic sp 2 carbon network locates near the Fermi level, it is reasonable that nitrogen species participate in the electrocatalytic reactions [36] , [37] . First-principle calculation based on density functional theory for elucidating the nature of the OER active site is now under investigation. In conclusion, the non-metal N/C electrocatalysts described here have the smallest overpotential for OER in alkaline solution and represent the first efficient non-metal electrocatalysts for the water-splitting reaction. We believe that our findings will facilitate the development of new families of OER electrocatalysts, because other heteroatoms, such as sulphur and boron, can be doped into the carbon matrix. Synthesis procedure of N/C and N/C–NiO x The procedure of N/C sample synthesis is displayed in Fig. 1 . In brief, melamine (6.45 g) was reacted with formaldehyde (12 ml, 37%) in 200 ml alkaline solution (1 g sodium hydroxide) at 80 °C for 4 h. After finishing the hydroxylation process, carbon particle (0.5 g, Ketjenblack EC-300J; Mistubishi Chemical) was dispersed in the above solution with an ultrasonic probe, followed by adding 20 ml hydrochloric acid (HCl) solution (pH 1) with 3.6 g Ni(NO 3 ) 2 ·6H 2 O. The pH value of the above solution was quickly tuned to pH 1 with concentrated HCl solution for 1 h polymerization. And then, NaOH solution (6 M) was added to tune pH 1–2 to form the polymer gel paste. The gel paste was dried in the oven under 150 °C for 5 h to crosslink the melamine formaldehyde resin. The solidated precursor was ground to powder using a Quartz mortar. Then, it was placed into a tubular furnace (Koyo) for pyrolysation at 700 °C in the presence of ammonia gas for 1.5 h. The N/C samples synthesized at the different temperatures are also pyrolysed in the presence of ammonia gas for 1.5 h. The prepared carbon mixture was ultrasonicly leached in concentrated HCl solution for 8 h to remove unbound metal species from the sample, and finished by distilled water washing and drying at 80 °C. The unleached sample, defined as N/C–NiO x , was ultrasonicly washed with distilled water and dried at 80 o C. Synthesis procedure of IrO 2 /C materials Synthesis of IrO 2 colloid was similar as a previous report [24] . K 2 IrCl 6 (0.1 g, 2.1 × 10 −4 mol) was added to 50 ml aqueous solution of 0.167 g of sodium hydrogen citrate sesquihydrate (6.3 × 10 −4 mol). The red-brown solution was adjusted to pH 7.5 with NaOH solution (0.25 M) and heated to 95 °C in an oil bath with constant stirring. After heating for 30 min, the solution was cooled to room temperature, and the NaOH solution was added to adjust the pH to 7.5. The addition of NaOH solution at room temperature, followed by heating at 95 °C for 30 min, was repeated until the pH value had stabilized at 7.5. The solution was transferred to a round-bottom flask with a reflux condenser. Then, 0.184 g carbon particle (KD-300J; Mistubishi Co.) was ultrasonically dispersed into the solution. The mixed solution was kept at 95 °C for 2 h with bubbled O 2 through the solution. The mixed IrO 2 /carbon solution was vacuum-dried at 70 °C. The IrO 2 /C (20 wt%) sample was heat-treated at 300 o C for 30 min to remove the organic compounds and washed with distilled water. Finally, the samples were collected by filtration and dried at 60 °C. Synthesis procedure of graphene/PDPS materials Graphene oxide was prepared by the Hofmann method [29] . Briefly, H 2 SO 4 (43 ml, 98%) and HNO 3 (14 ml, 68%) were added to a reaction flask cooled by immersion in an ice bath. Graphite (2 g, Aldrich Co.) was then added into the acid mixture with stirring to achieve the uniform dispersion. KClO 3 (25 g) was slowly added to the above mixture in an ice bath and stirred for 3 days at room temperature. After finishing the reaction, 3 l water was pulled into the flask. Graphite oxide was collected by filtration and redispersed in HCl (5%) solutions to remove sulphate ions. Graphite oxide slurry was then dried in a vacuum oven at 0 o C for 48 h before use. PDPS (0.4 g) (ref. 30 ) and graphene oxide (0.6 g) were mixed in 10 ml dimethylsulphoxide and ultrasonically dispersed for 30 min. The mixture was stirred at 100 °C for 1 h, and the solvent was removed using a rotary evaporator. The graphene oxide/PDPS was pulverized using a quartz mortar. For the pyrolysed sample, the graphene oxide/PDPS material was put into the bottom of a half-closed quartz tube in argon atmosphere. The tube was quickly inserted into a muffle furnace preheated to 900 °C, and graphene oxide/PDPS material was pyrolysed for 5 min. After heat treatment, the tube was quickly removed from the furnace and cooled under argon flow to yield the pyrolysed graphene/PDPS sample. Commercial Pt/C (20 wt%) was purchased from Tanaka Kikinzoku. Physical characterization The XRD of the samples was analysed using an XRD analyser (Panarytical PW-1700; Spectris). SEM was performed using a SU-8000 machine (Hitachi). TEM was carried out using a H-9000UHR machine (Hitachi; 300 kV). A Micromeritics Tristar 3000 machine (Shimadzu) was used to measure Brunauer–Emmett–Teller surface area. XPS was performed to analyse surface elemental composition, in which a Kratos Ultra AXIS Spectrometer system equipped with a monochromatic Al-Kα source (15 kV). The amount of the evolved oxygen in KOH electrolyte (pH 13) was monitored simultaneously with the positive potential scan tests using a needle-type oxygen microsensor (Microx TX3-trace; Presens). The electrical resistivity of the N/C materials was measured with a four-probe method by Loresta-GP T610 (Mistubishi). Elemental analyses of possible metal species in the N/C samples were also conducted using an ICP-AES (ICPS-8000; Shimadzu). Electrode preparation and characterization The OER activities were measured using a bipotentiostat (Pine Instrument Co.) equipped with a RRDE. A SCE was used as the reference electrode in the bipotentiostat measurement RRDE system and was calibrated with respect to a RHE (RHE=SCE*+0.244 V+0.591 × pH at 25 °C). A glassy carbon disk (0.2 cm −2 ) and Pt wire were used as the working and counter electrodes, respectively. In the RRDE system, the working electrode was prepared by loading catalyst ink (0.2 mg cm −2 ; a mixture of 2 mg catalyst, 5 μl Nafion solution (5 wt%; DuPont) and 1 ml ethanol) on the glassy carbon electrode. RRDE measurements were conducted in an oxygen-saturated KOH solution (pH 13) at 25 °C using a scan rate of 5 mV s −1 and a rotation speed of 1,500 r.p.m. (Pine Instrument Co.). Before performing the RRDE experiments, the Pt ring was activated by potential cycling several times between 0.1 and 1.4 V in 0.05 M H 2 SO 4 . The poisoned potential on the Pt ring is 1.51 V versus RHE. Calculation of the EASA The EASA of bare glassy carbon disk electrode was calculated using the following equation [38] : where n is the number of electrons transferred (ferrocyanide, n =1), F is Faraday’s constant (96,485 C mol −1 ), R is the gas constant (8.314 J mol −1 K −1 ), T is the temperature (298 K) and C R * (mol l −1 ) is the initial ferrocyanide concentration and v is the CV scan rate (0.05 V s −1 ). The diffusion coefficient ( D R ) of ferrocyanide was based on the reference data (3.7 × 10 −6 cm 2 s −1 ) (ref. 38 ), and the calculated surface area of bare glassy carbon disk electrode is 0.2 cm 2 . This value is well consistent to the data supported by the company (0.198 cm 2 ). The EASA of the porous N/C electrodes was calculated using double-layer capacitor with following equation [39] , [40] : where ε r is the electrolyte dielectric constant, ε 0 is the dielectric constant of the vacuum, d is the effective thickness of the double layer (charge separation distance), A is the EASA, I is the response current density, V is the potential (V), t is the potential scan rate and m is the mass of the N/C composite in the electrodes. The CV diagrams with different amounts of N/C catalysts on the glassy carbon electrode (RRDE system) and the relationship between the capacitor and loaded catalyst amounts were plotted in Supplementary Fig. S10 . It can be confirmed that the capacitors of N/C electrodes showed linear relationship with their EASA. Based on equation (2), the EASA of porous N/C electrode can be calculated based on A 1 /A 2 =C 1 /C 2 (A 1 is glassy carbon electrode, 0 mg cm −2 , 0 mg; A 2 is the N/C catalyst electrode, 2 mg cm −2 , 0.04 mg). EASA of the N/C electrode (0.2 mg cm −2 (GSA, 0.2 cm 2 )) was calculated to be 17.5 cm 2 . Similar calculations were performed for all of other N/C catalysts. Evaluation of the OER activity of the N/C materials We used the ICP-AES to detect the possible trace amount of metal species in the N/C materials. The limited detection of the used ICP-AES was as low as 0.001 at%. The detected concentration of nickel was 0.002 at%. We hypothesized that all of nickel species were active for OER and calculated the turnover frequency (TOF) based on the observed OER currents and 0.002 at% metal species. At a potential of 1.58 V (versus RHE), the current exhibited by N/C—700 o C electrode was 1.32 × 10 −3 A (read directly from RRDE data). The EASA of the N/C electrode was 17.5 cm 2 . The BET surface area of N/C—700 o C catalysts was 560 m 2 g −1 . The used catalyst amount on the electrode was 4 × 10 −5 g. N A was Avogadro constant. The percentage of the evolved catalysts on the N/C electrode: (17.5 cm 2 /560 m 2 g −1 × 4 × 10 −5 g)=8%. The content of metal species was 0.002 at%. The amount of catalyst was 4 × 10 −5 g/12 g mol −1 =3.3 × 10 −6 mol. Then, we determinate the active metal species on the surface of our sample: =3.3 × 10 −6 mol × 8% × 0.002% × N A =5.3 × 10 −12 N A atoms. The TOF at 1.58 V versus RHE (current, 1.32 × 10 −3 A)=((1.32 × 10 −3 A) N A )/96,485.3/(5.3 × 10 −11 N A )=2,600 s −1 . Based on the above calculation, TOF of the N/C materials based on 0.002 at% of nickel species was 2,600 s −1 . As reported previously, the well-known cobalt oxide showed the highly efficient OER activities with the TOF range from 0.01–2 s −1 at the potential of 1.58 V versus RHE [2] . One of the best cobalt oxide OER electrocatalysts (CoO x /Au) was reported to show the high TOF (at 1.58 V, 1.8 s −1 ) (ref. 2 ). Compared with the TOF of CoO x /Au, the TOF of the N/C materials based on 0.002 at% nickel species (2,600 s −1 ) was unreasonable. On the basis of the calculation, it can be concluded that the high OER current generated from the N/C materials should be from the nitrogen-related active sites. How to cite this article: Zhao, Y. et al . Nitrogen-doped carbon nanomaterials as non-metal electrocatalysts for water oxidation. Nat. Commun. 4:2390 doi: 10.1038/ncomms3390 (2013).